Adaptation in bacterial CRISPR-Cas immunity can be driven by defective phages Clustered regularly interspaced short palindromic repeats (CRISPRs) and their associated cas genes serve as a prokaryotic ‘adaptive’ immune system, protecting against foreign DNA elements such as bacteriophages. CRISPR-Cas systems function by incorporating short DNA ‘spacers’, homologous to invading DNA sequences, into a CRISPR array (adaptation). The array is then transcribed and matured into RNA molecules (maturation) that target homologous DNA for cleavage (interference). It is unclear how these three stages could occur quickly enough in a naive phage-infected cell to interfere with phage replication before this cell would be irrevocably damaged by the infection. Here we demonstrate that cells can acquire spacers from defective phages at a rate directly proportional to the quantity of replication-deficient phages to which the cells are exposed. This process is reminiscent of immunization in humans by vaccination with inactivated viruses. Clustered regularly interspaced short palindromic repeats (CRISPR) and their associated cas genes [1] serve as a prokaryotic ‘adaptive’ immune system, protecting against foreign DNA elements such as bacteriophages [2] and plasmids [3] . This immunity is conferred by site-specific cleavage of the invading DNA element, targeted by short DNA ‘spacers’ present in the CRISPR array and homologous to the invading sequence. The remarkable ability to acquire new specificities by incorporating additional spacers is what sets CRISPR-Cas systems apart from other, analogous, microbial defense systems [4] . Genetic manipulation of the arrays has also enabled their use as targeted genome editing tools, a field which has exploded in 2013 (ref. 5 ). However, the process of natural spacer acquisition remains enigmatic, demonstrated in the laboratory in only a few systems [2] , [6] , [7] , [8] , [9] . In contrast, acquisition of spacers is clearly occurring in natural populations, which diverge considerably at their CRISPR loci [10] , [11] . Streptococcus thermophilus possesses two active type II-A CRISPR systems [12] (CR1 and CR3) and is by far the best-studied model of natural spacer acquisition. This is due, at least partly, to the negligible frequency of phage resistance by mechanisms other than CRISPR-Cas. Bacteriophage-insensitive mutants (BIMs) in this bacterial species are almost always associated with spacer acquisition in either the CR1 and/or CR3 arrays [12] , [13] . To our knowledge, the process of acquiring CRISPR-based immunity against phages in this system requires phage infection of the host cell and concomitant exposure to the phage double-stranded DNA genome followed by spacer acquisition (adaptation [14] ), expression and maturation of the newly acquired spacer to generate ‘targeting’ crRNA molecules (maturation [15] ) and, only then, cleavage of the invading DNA (interference [3] , [16] ). It is difficult to imagine all of these steps occurring before the accumulation of lethal damage to the cell from an invading virulent phage. One of the existing hypotheses [17] addressing this conundrum is that the majority of spacer acquisition happens on infection by a defective phage, either incapable of replication or significantly delayed in its ability to damage the host cell beyond recovery. These phages could be defective because of some inherent flaw: mutations, DNA damage, faulty packaging of their genome—or because of interference by the host inactivating them shortly after the genome enters the cell. Here we demonstrate that the presence of defective phages, whether inherently so or generated by another host defense mechanism, greatly favours the emergence of CRISPR-based immunity. Generating defective phages We first generated a ‘defective’ phage using a restriction-modification (RM) system, LlaDCHI [18] , [19] , which has already been shown to be compatible with the CRISPR-Cas system in S. thermophilus [20] . LlaDCHI is a type II RM system similar to DpnII, which cleaves the double-stranded unmethylated sequence 5′-GATC-3′. 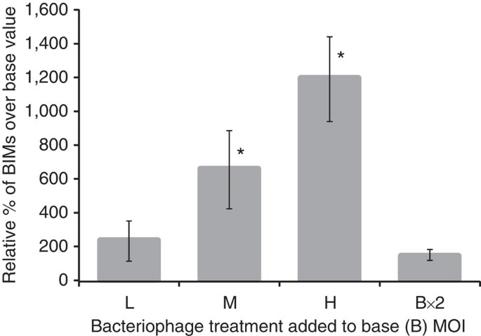Figure 1: Bacteriophage-insensitive mutant count on exposure to defective phages. The average ratio of the number of BIMs from each treatment (L, M, H, B × 2) over the number of BIMs in the control within that biological replicate. The BIM counts are the average number of colonies obtained from three technical replicates for each of three independent biological replicates on exposure to phages at a base MOI of 0.1 of 2972M+, plus either a Low (L, 0.01), Medium (M, 0.05) or High (H, 0.10) MOI of ‘defective’ 2972 wild-type phage, or, as a control, an additional MOI of 0.1 of 2972M+ (B × 2). Error bars represent the s.d. of the average ratios. *Significant difference (P<0.01) from all other treatments, as determined by linear mixed-effects analysis of variance (R package: lme4: linear mixed-effects models using S4 classes. v. 0.999999-0) and Tukey’s honest significant difference30. When the wild-type virulent phage 2972 is first plated on the S. thermophilus RM+ strain SMQ-1279 (see Construction of S. thermophilus RM and control strains in Methods), a derivative of the wild-type phage-sensitive host S. thermophilus DGCC7710, it suffers a 5-log reduction in efficiency of plating (EOP) ( Table 1 ). This reduction is due to the cleavage of GATC sites in the phage genome by the endonuclease LlaDCHI-C [20] . Phages recovered from rare productive infections yielded phages with a methylated genome (M+) to escape cleavage by the RM system. These 2972M+ phages re-plated on the RM-containing strain SMQ-1279 resulted in titres comparable to that of the wild-type 2972 plated on its host DGCC7710 ( Table 1 ). When these 2972M+ phages were titred on the wild-type strain, their titres were also similar (within 1%) to those obtained on SMQ-1279 ( Table 1 ). Effectively, we had a ‘functional’ phage, 2972M+, and, when plated on SMQ-1279, a readily titrable ‘defective’ phage: the wild-type 2972. Table 1 Treatments and EOP of phages in this study. Full size table Inherently defective phages were also obtained by exposing the same 2972M+ phages to ultraviolet radiation. Four different ultraviolet treatments were used, varying in time (2.5, 5 or 10 min) or intensity (L, low; H, high) leading to either a reduction of 4 logs in functional phages (UV10(L), UV2.5(H)) or their complete inactivation (UV5(H), UV10(H), EOP <10 −8 ) ( Table 1 ). BIM assays BIM assays were performed by challenging S. thermophilus SMQ-1279 with phage 2972M+ at a base (B) multiplicity of infection (MOI) of 0.1 plaque-forming units per colony-forming unit (~10 7 plaque-forming units per 10 8 colony-forming units), sufficient to maintain selective pressure by killing phage-sensitive cells and allow growth of BIM colonies. In addition to this base (B) MOI, the cells were also exposed to a low (L=0.01), medium (M=0.05) or high (H=0.1) MOI of unmethylated ‘defective’ phages 2972, or, as a control, an additional 0.1 MOI (B × 2=0.2) of functional 2972M+. The addition of the defective phages led to a consistent increase in the number of BIMs relative to the base value ( Fig. 1 ), rising to over tenfold at the highest MOI of defective phages. In contrast, doubling the number of functional phages (B × 2, an MOI of 0.2 functional phages) to match the highest total phage count used (H, with an MOI of 0.1 functional and 0.1 defective phages.) had no significant effect on the number of BIMs generated. PCR assays confirmed that the resulting BIMs contained a new spacer at either CRISPR 1 (90%) or CRISPR 3 (7%) (3% PCR failure). Figure 1: Bacteriophage-insensitive mutant count on exposure to defective phages. The average ratio of the number of BIMs from each treatment (L, M, H, B × 2) over the number of BIMs in the control within that biological replicate. The BIM counts are the average number of colonies obtained from three technical replicates for each of three independent biological replicates on exposure to phages at a base MOI of 0.1 of 2972M+, plus either a Low (L, 0.01), Medium (M, 0.05) or High (H, 0.10) MOI of ‘defective’ 2972 wild-type phage, or, as a control, an additional MOI of 0.1 of 2972M+ (B × 2). Error bars represent the s.d. of the average ratios. *Significant difference ( P <0.01) from all other treatments, as determined by linear mixed-effects analysis of variance (R package: lme4: linear mixed-effects models using S4 classes. v. 0.999999-0) and Tukey’s honest significant difference [30] . Full size image Using a similar BIM assay but with a different type of defective phage, an estimated MOI of 0.1 of ultraviolet-defective phages, the number of BIMs increased by three- to fourfold significantly, although not as efficiently as with the RM system ( Fig. 2 ). This lower efficacy is probably due to the inability of some ultraviolet-treated phages to inject their DNA, as evidenced by the failure of the most harshly ultraviolet-treated (UV10(H)) phages to augment the number of BIMs. It was of particular interest that the addition of UV5(H)-treated phage lysate, which contained no functional phage, still led to a significant increase in the number of BIMs through spacer acquisition. 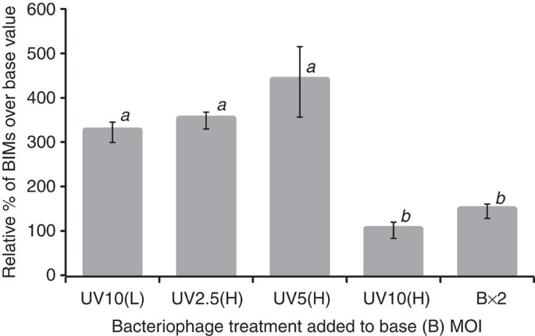Figure 2: Bacteriophage-insensitive mutant counts on exposure to ultraviolet-treated phages. The average ratio of the number of BIMs from each treatment over the number of BIMs in the control within that biological replicate. The BIM counts are the average number of colonies obtained from three technical replicates for each of three independent biological replicates on exposure to phages at a base MOI of 0.1 of 2972M+, plus an equal volume of either ultraviolet-treated phages (seeTable 1) or, as a control, an additional MOI of 0.1 of 2972M+ (B × 2). Error bars represent the s.d. of the average ratios. All samples markedaare significantly different (P<0.05) from those markedb, as determined by one-way analysis of variance and Tukey’s honest significant difference30. Figure 2: Bacteriophage-insensitive mutant counts on exposure to ultraviolet-treated phages. The average ratio of the number of BIMs from each treatment over the number of BIMs in the control within that biological replicate. The BIM counts are the average number of colonies obtained from three technical replicates for each of three independent biological replicates on exposure to phages at a base MOI of 0.1 of 2972M+, plus an equal volume of either ultraviolet-treated phages (see Table 1 ) or, as a control, an additional MOI of 0.1 of 2972M+ (B × 2). Error bars represent the s.d. of the average ratios. All samples marked a are significantly different ( P <0.05) from those marked b , as determined by one-way analysis of variance and Tukey’s honest significant difference [30] . Full size image Source of the acquired resistance We performed a complete ultraviolet inactivation of the virulent phage 858 (ref. 21 ), which is 90.9% identical to phage 2972 at the nucleotide level, shares many potential CRISPR targets and can infect the same host strain. We first exposed the cells to the completely ultraviolet-inactivated 858 phages (ultraviolet-858) for 4 h at an estimated MOI of 5. We then challenged these 858-exposed cells with functional 2972M+ phages (MOI of 0.1) to select for BIMs (spacer acquisition). An ~6-fold increase in BIM formation was observed relative to the control cells exposed to only functional 2972M+ phages ( Table 2 ). We compared the spacer sequences acquired by the BIMs in this challenge with those obtained from phage 2972 treatments described in Figs 1 and 2 ( Table 2 ). As expected, nearly 100% of the acquired spacers perfectly matched the genome of the phage used for BIM selection, 2972M+. When obtained from exposure to solely 2972M+, only a third of these spacers also matched phage 858’s genome. By comparison, of the spacer sequences obtained following the double challenge (defective 858 followed by 2972M+), 87.2% of them matched both phage genomes, suggesting acquisition primarily from the defective 858 phages. Furthermore, one of the acquired spacers matched the genome of phage 858 perfectly, but not that of 2972. The spacer’s sequence (5′-GAAGTATTA A GTCTCTCAAAAGATGATATT-3′) differs from a 2972 proto-spacer by a G->A substitution (base in bold type). The spacer still confers resistance to phage 2972 despite the single mismatch, but was clearly acquired from a defective phage 858. Table 2 Comparison of BIM sequences targeting phages 2972 and 858. Full size table Here we showed that exposure to defective phages, whether because of interference by the host or because of flaws in the virion, greatly favoured spacer acquisition in CRISPR-based immunity ( Figs 1 and 2 ). When exposed to unmethylated phage, the rate of resistance acquisition increased as the titre of unmethylated phages used increased. Notably, in treatments with the same total number of phage particles (for example, H and B × 2), acquisition of immunity was greatly favoured in the presence of defective particles. Clearly, exposure to defective phages greatly increases spacer acquisition in such a way that additional functional phages do not. Testing our defective phage hypothesis with an RM system was advantageous for a number of reasons: it allowed precise knowledge of the number of additional defective phages by titre on a permissive host; it confirmed that these phages are defective only once the DNA is present inside the host rather than deficient in adsorption, attachment or penetration, all of which would prevent the host cell from being exposed to phage DNA; and it resulted in a high proportion of defective phages. An alternative might have been to expose an already CRISPR-immune BIM to phages against which it carries a spacer. However, this would have been complicated by the posited role of ‘priming’ in spacer acquisition [22] , [23] , a process by which previous spacer acquisition can increase acquisition even when the spacer is not sufficiently homologous to the invading phage to confer immunity. Extending our findings to ‘inherently’ defective phage, inactivated by ultraviolet treatment and therefore defective before contact with the host, proved particularly useful despite the inability to precisely quantify them. First, obtaining similar increases in BIM generation through spacer acquisition allowed us to confirm this property was linked to the presence of defective phages and was not an artefact of RM-mediated interference. Second, the ability to obtain 100% defective phage for another phage–host pairing allowed us to convincingly demonstrate that spacers were being acquired from the defective phages themselves. As spacers can be acquired from the genome of defective phages, it is tempting to suggest that the acquisition rate from ‘functional’ phages is due to some percentage of defective phages already present in the total phage population of a lysate. Alternatively, the naive CRISPR-Cas system itself might be responsible for generating some defective phages before acquisition-based immunity. To test this hypothesis, we titred the wild-type 2972 phages on a S. thermophilus strain deficient in interference, SMQ-1143 (DGCC7710:: pcas9- ) [3] . The phage titres were indistinguishable from those on the wild-type strain ( Table 1 ), leaving us with no reason to suppose that the defective phages are generated by the naive CRISPR-Cas system itself. We propose a model in which we assume that the phage 2972M+ lysate contains 10% inherently defective phages, and, therefore, that the addition of an MOI of 0.01 (L) of 2972 to an MOI of 0.1 of 2972M+ is doubling the number of defective phages. Applying this assumption to data obtained with the RM system ( Fig. 1 ) results in a convincing almost 1:1 correlation between the relative change in defective phages and the change in relative BIM counts ( Fig. 3 ). Furthermore, this would attribute >96% of BIMs to defective phages (X intercept, where defective phage count=0, resistance=3.4%). This is consistent with the notion that all acquisition of CRISPR immunity is due to exposure to defective phages. The sensitivity and relative accuracy of current techniques for counting functional (plaque assays) and defective viral particles (Nanosight, quantitative PCR, electron microscopy and epifluorescence microscopy) lack the accuracy required to test this hypothesis [24] . More importantly, these techniques would be unable to distinguish between phages defective for replication and those deficient upstream of the DNA injection process, which presumably do not interact with the CRISPR-Cas system at all. 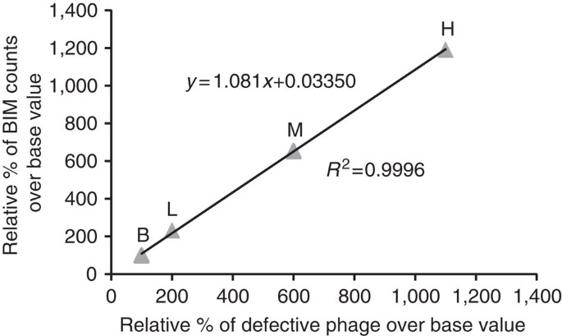Figure 3: Prediction of a direct correlation between relative change in BIM counts and relative change in defective phage. The model assumes only that the base (B) treatment includes 10% defective phages and that the correlation is linear. The data were obtained fromFig. 1, where the % of defective phage is relative to the assumed value in the base (B) treatment. Figure 3: Prediction of a direct correlation between relative change in BIM counts and relative change in defective phage. The model assumes only that the base (B) treatment includes 10% defective phages and that the correlation is linear. The data were obtained from Fig. 1 , where the % of defective phage is relative to the assumed value in the base (B) treatment. Full size image Taken altogether, our data clearly show that when defective phages are present, they are responsible for the vast majority of the acquisition of CRISPR-mediated phage immunity. Although we cannot convincingly attribute all spacer acquisition events to defective phages, our data helps explain the apparent difficulties in the timing of immunity acquisition. They might also explain some of the discrepancies in acquisition between phage–host systems, each with a different proportion of defective phages. The widely applicable nature of ultraviolet inactivation for other phages may allow the detection of adaptation in CRISPR-carrying organisms not yet shown to acquire new spacers. This will serve not only to increase the scope of CRISPR research, but should facilitate the generation of phage-resistant strains for bioprocesses susceptible to disruption by phages. In fact, this immunity gained from defective phages can be likened to vaccination of humans against a virus with high morbidity. By exposure to a ‘safe’, attenuated or inactivated form of the virus, the host is given the opportunity to acquire immunity. Construction of pORI28-derived plasmids To integrate the LlaDCHI RM system into S. thermophilus DGCC7710 (ref. 25 ), the RM system was first cloned into the Gram-positive suicide vector pORI28 (ref. 26 ). To do so, plasmid pSRQ707 containing the LlaDCHI system [19] was digested with EcoRV and NruI, and the fragment containing the RM system was purified before being ligated to the EcoRV-linearized pORI28. Ligation products were then transformed into Escherichia coli EC1000 cells (MC1000 RepA+, Km R ) and one pORI:LlaDCHI clone was selected and confirmed by sequencing. We elected to integrate the LlaDCHI system into a putative α-amylase encoding gene ( amyL , stu1542 in S. thermophilus LMG 18311), which we found through BLAST searches on the S. thermophilus DGCC7710 genome sequence. We hypothesized that inactivating this gene would not interfere with any defense system of the host. An internal part (481 bp, position 217–697) of the gene (1,476 bp) was amplified by PCR using primers MV-amylRD-39F-EcoRI and MV-amylRD-672R-BglII ( Table 3 ). The PCR product was digested with EcoRI and BglII, purified and ligated into the digested pORI:LlaDCHI clone. Following transformation into E. coli EC1000 cells, several clones were obtained after 5 days of incubation at 37 °C on selective medium. Selected clones containing the construct pORI:LlaDCHI-amyl were all confirmed by sequencing. Table 3 Primers used in the study. Full size table We also digested the pORI:LlaDCHI-amyl construct with XbaI and NheI, and the fragment containing pORI28 with the gene fragment was religated on itself (pORI:amyl) before transformation into E. coli EC1000. Construction of S. thermophilus RM and control strains The pORI:LlaDCHI-amyl construct was transformed into S. thermophilus DGCC7710 through its natural competence [27] . Competent cells were prepared using chemically defined medium (CDM) [28] . S. thermophilus DGCC7710 cells were grown overnight at 37 °C without shaking in liquid LM17 medium (consisting of M17 (Oxoid, Ontario, Canada) with 0.5% w/v lactose), washed with CDM medium at room temperature and the cell pellet was resuspended in an equal volume of fresh CDM medium. The culture was diluted 30-fold and incubated at 37 °C before adding the competence-inducing octapeptide ComS17-24 (>97% purity, Peptide 2.0) [27] to a final concentration of 1 μM alongside 5 μg purified plasmid pORI:LlaDCHI-amyl to 300 μl of cells, and then incubated again for 3 to 4 h at 37 °C. Aliquots of the mixtures were plated on selective media (LM17 containing 3 μg ml −1 erythromycin) and incubated in anaerobic jars for at least 24 h at 37 °C. Clones were then checked for integration into the amylase gene by PCR using one flanking primer (MV-RDAmyl-1409Rev) and an internal primer (MV-Lla1R) ( Table 3 ). PCR products were sequenced to confirm integration. The selected clone was named S. thermophilus SMQ-1279 (DGCC7710 amyl :pORI-LlaDCHI, Em R ). Inactivation of the amylase gene was done as above, but by using the pORI:amyl plasmid. Clones were obtained following natural transformation of competent DGCC7710 cells and integration of pORI:amyl into the amylase gene was confirmed by PCR and sequencing. Primers used were pORIRev (as an internal primer) and MVamyl1409R ( Table 3 ). A selected clone was named SMQ-1280 (DGCC7710 amyl : pORI28, Em R ). Phage 2972 had an EOP of 1.0 on SMQ-1280, similar to that on the parent DGCC7710, confirming the inactivation of the amylase gene has no impact on phage replication. Obtaining methylated phage 2972 Phage 2972M+ was obtained by passage of wild-type phage 2972 (ref. 25 ) on SMQ-1279 in LM17-CaCl medium (consisting of LM17 supplemented with 10 mM CaCl 2 ), purification from a single plaque and subsequent enrichment by amplification on SMQ-1279, followed by 0.45 μm filtration of the lysate and storage at 4 °C. Methylation of the phage genome was confirmed by restriction digest of the purified phage genomic DNA with DpnI. Phage titres and EOP Overnight cultures were used to inoculate at 1% LM17 broth cultures grown at 42 °C until they reached an OD 600 (optical density) of 0.6. Next, 500 μl of culture and 100 μl of serially diluted phage lysate in phage buffer (50 mM Tris-HCl, pH 7.5, 100 mM NaCl, 8 mM MgSO 4 ) were added to 3 ml of molten LM17-CaCl 0.75% w v −1 agar, mixed briefly, and pour atop an LM17-CaCl 2 1% agar plate without selection. Plates were incubated at 42 °C in a sealed bag for 24 h, then plaques were counted. EOP was determined by dividing the phage titre obtained on the resistant strain by the phage titre obtained on the wild-type strain. Phage MOIs and culture ODs used in this study were chosen to increase reproducibility. BIM counts were found to be higher at greater MOIs and an OD 600 of 0.8, resulting in frequencies of ~1E−06, but they were also more variable. Ultraviolet treatments for phage inactivation Five hundred microlitres of 2972M+ or 858 lysate was spread out on a plastic petri plate, and spread evenly over either 9 cm 2 (depth of 520 μm or (L) treatment) or 16 cm 2 (depth of 313 μm or (H) treatment). The plates were then placed on a ultraviolet sterilizer (Millipore, Cat XX6370000) at a distance of 12 cm from TUV8W/G8T5 bulbs for 2.5, 5, 6 or 10 min. The samples were recovered by pipetting, titred and used for BIM assays. The amplification of ultraviolet-inactivated 858 (6 min) on the sensitive host resulted in no detectable plaques (<10 phages per ml) confirming complete inactivation ( Table 1 ). BIM assays Phage lysates were diluted in phage buffer to obtain a calculated MOI of phages 2972M+ plus a calculated MOI of phage 2972, or an estimated MOI of ultraviolet-treated phages 2972 or 858. Phage and culture combinations were plated as for phage titres, and the number of phage-resistant colonies were counted after 24 h. Ten colonies were picked for each MOI tested, grown overnight in 1 ml LM17 with selection and 2 μl used as a template for PCRs to confirm, by size of product, the acquisition of spacers [29] CRISPR loci 1 and 3. A total of 100 BIM colonies were so screened. In addition, 181 such CRISPR locus 1 PCR products (not pre-screened for acquisition) were sequenced to determine the sequence of the acquired spacer ( Table 2 ). How to cite this article: Hynes, A. P. et al. Adaptation in bacterial CRISPR-Cas immunity can be driven by defective phages. Nat. Commun. 5:4399 doi: 10.1038/ncomms5399 (2014).